Multiple pore conformations driven by asynchronous movements of voltage sensors in a eukaryotic sodium channel Voltage-dependent Na + channels are crucial for electrical signalling in excitable cells. Membrane depolarization initiates asynchronous movements in four non-identical voltage-sensing domains of the Na + channel. It remains unclear to what extent this structural asymmetry influences pore gating as compared with outwardly rectifying K + channels, where channel opening results from a final concerted transition of symmetric pore gates. Here we combine single channel recordings, cysteine accessibility and voltage clamp fluorimetry to probe the relationships between voltage sensors and pore conformations in an inactivation deficient Nav1.4 channel. We observe three distinct conductance levels such that DI-III voltage sensor activation is kinetically correlated with formation of a fully open pore, whereas DIV voltage sensor movement underlies formation of a distinct subconducting pore conformation preceding inactivation in wild-type channels. Our experiments reveal that pore gating in sodium channels involves multiple transitions driven by asynchronous movements of voltage sensors. These findings shed new light on the mechanism of coupling between activation and fast inactivation in voltage-gated sodium channels. Voltage-gated ion channels are biological equivalents of transistors for propagating and amplifying electrical signals in excitable cells [1] , [2] . These proteins consist of a central ion conducting pore and four discrete voltage-sensing domains, which together give rise to a conductance even more steeply voltage-dependent than their silicon-based counterparts [3] . Much of our present knowledge about the gating mechanisms of this family of ion channels comes from studies on voltage-dependent potassium channels, which derive their steep voltage dependence by requiring that pore opening be a single concerted step following activation of four identical voltage-sensing domains [4] , [5] , [6] , [7] . However, unlike potassium channels, eukaryotic sodium and calcium channels consist of four asymmetric domains DI-IV, which raise questions about the conserved nature of the gating transitions in these channels. Sodium channels rapidly inactivate after opening, which helps reset the membrane for the next electrical impulse. Although fast inactivation results from pore occlusion by a hydrophobic motif [8] , [9] , [10] , disease-causing mutations throughout the channel affect fast inactivation, suggesting that this process is intimately coupled to global conformational changes [11] , [12] , [13] , [14] , [15] , [16] , [17] . In particular, studies with fluorescent probes [18] , gating modifier toxins [19] , mutagenesis [11] , [15] , [20] , [21] and paddle chimeras [22] imply that whereas DI-III are primarily involved in activation, DIV has a distinct role in inactivation. However, the mechanism underlying this relationship between DIV movement, channel opening and inactivation remains poorly understood. The development of well-constrained detailed kinetic models for sodium channel activation has been hindered by fast inactivation, which typically masks all but the first few channel-opening events [23] . Although various toxins or proteases impair fast inactivation, possible nonspecific effects of these compounds make it difficult to interpret apparently conflicting results, such as whether or not activation and fast inactivation overlap [24] , [25] , [26] , [27] . Thus, removing inactivation by protein engineering represents an attractive approach to study the activation process in isolation, and has been used to develop quantitative models of Shaker potassium channel activation [4] , [5] , [6] . The mutations I1488Q/F1489Q/M1490Q (QQQ) in the DIII-IV linker [8] , or L435W/L437C/A438W (WCW) in the DI-S6 segment [28] , each largely remove fast inactivation in voltage-gated sodium channels, possibly by disrupting the inactivation motif or its access to its docking site, respectively. However, the QQQ mutant expresses poorly in heterologous systems, whereas Nav1.4-WCW expresses sufficiently well for single channel studies. Furthermore, Nav1.4-WCW has little effect on the macroscopic current–voltage relation [28] or binding affinity for local anaesthetics such as lidocaine [29] , suggesting that this mutant may be a good model for studying activation in isolation from fast inactivation. Here we combined single channel recordings, cysteine accessibility, and fluorescence measurements from site-specific probes to study activation gating in a fast inactivation-deficient mutant Nav1.4-WCW. Our observations reveal that sodium channel pore opening involves at least two steps, where the initial opening corresponds to activation of DI-III voltage sensors, and subsequent activation of the DIV voltage sensor initiates formation of a distinct subconducting pore conformation, which not only precedes, but is also the rate-limiting step for fast inactivation. These data imply that activation of the DIV voltage sensor does not directly promote fast inactivation, but instead induces a conformational change of the pore necessary for fast inactivation to occur. The WCW mutations severely impair fast inactivation Responses to depolarizing voltage steps were recorded from HEK293 cells expressing rat Nav1.4 or Nav1.4-WCW channels. Nav1.4-WCW capacitance-normalized whole-cell currents were three-fold larger than for Nav1.4 ( t -test, P <0.001). Nav1.4 currents inactivated nearly completely within 5–10 ms, whereas Nav1.4-WCW did not show appreciable inactivation during the 20 ms test pulse ( Fig. 1a ). Nav1.4-WCW current rise was prolonged compared with Nav1.4 at hyperpolarized potentials, but approached that of Nav1.4 at depolarized potentials ( Supplementary Fig. S1a,b ). Although the extrapolated delay in current onset t 0 following the voltage step is contaminated by the time required to charge the cell membrane, the similar delay for Nav1.4 and Nav1.4-WCW imply that any differences must be less than t 0 ( Supplementary Fig. S1c ). 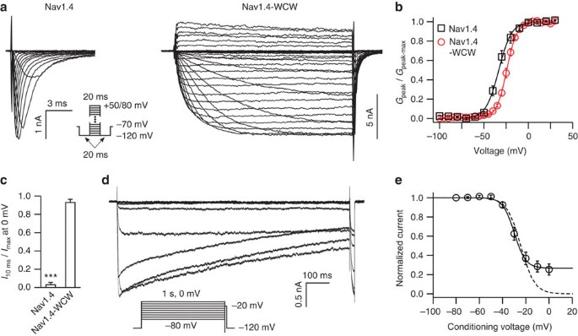Figure 1: Nav1.4-WCW severely disrupts fast inactivation and eliminates inactivation from closed states. (a) Whole-cell current responses to 20 ms depolarizing voltage steps for rat Nav1.4 (left, only 10 ms shown) and rat Nav1.4-WCW (right) channels at room temperature. Cells were held at −70 mV and hyperpolarized to −120 mV for 20 ms before and following a 20 ms depolarizing pulse from −120 to +50 mV (Nav1.4) or +80 mV (Nav1.4-WCW) in 5–10 mV steps (see inset). (b) Normalized peak conductance–voltage (G–V) relation from recordings as shown ina(mean±s.e.m.). The voltage at which the conductance was half maximal (V1/2) and the effective charge (z) from single Boltzmann fits to the G–V from individual cells were, for Nav1.4 (mean±s.e.m.):V1/2=-32.6±1.9 mV,z=3.8±0.4 e−,n=5; and for Nav1.4-WCW:V1/2=-24.9±0.8 mV,z=4.7±0.2 e−,n=8. Single Boltzmann fits to the mean were for Nav1.4:V1/2=-33.3 mV,z=3.4 e−, and for Nav1.4-WCW:V1/2=-24.4 mV,z=4.2 e−. (c) Summary of the fraction of the peak current remaining after 10 ms for Nav1.4 and Nav1.4-WCW (mean±s.e.m.). ***t-Test,P<0.001. (d) Nav1.4-WCW whole-cell current responses to a steady-state inactivation protocol consisting of a 20 ms test pulse to −20 mV to assay the fraction of available (that is, non-slow inactivated) channels after a 1 s preconditioning pulse from −80 to 0 mV at room temperature (see inset). Holding potential was –120 mV and a 1 ms hyperpolarizing pulse to −140 mV preceded each test pulse. (e) The normalized peak current response during the test pulse is plotted against the voltage during the preconditioning pulse for five cells (open circles, mean±s.e.m.,n=5) fit with a single Boltzmann plus an added constant (solid line;V1/2=-29.9 mV,z=4.9 e−, constant=0.27). The G–V relation for Nav1.4-WCW frombis shown inverted for comparison (dashed line). Figure 1: Nav1.4-WCW severely disrupts fast inactivation and eliminates inactivation from closed states. ( a ) Whole-cell current responses to 20 ms depolarizing voltage steps for rat Nav1.4 (left, only 10 ms shown) and rat Nav1.4-WCW (right) channels at room temperature. Cells were held at −70 mV and hyperpolarized to −120 mV for 20 ms before and following a 20 ms depolarizing pulse from −120 to +50 mV (Nav1.4) or +80 mV (Nav1.4-WCW) in 5–10 mV steps (see inset). ( b ) Normalized peak conductance–voltage (G–V) relation from recordings as shown in a (mean±s.e.m.). The voltage at which the conductance was half maximal ( V 1/2 ) and the effective charge ( z ) from single Boltzmann fits to the G–V from individual cells were, for Nav1.4 (mean±s.e.m. ): V 1/2 =-32.6±1.9 mV, z =3.8±0.4 e − , n =5; and for Nav1.4-WCW: V 1/2 =-24.9±0.8 mV, z =4.7±0.2 e − , n =8. Single Boltzmann fits to the mean were for Nav1.4: V 1/2 =-33.3 mV, z =3.4 e − , and for Nav1.4-WCW: V 1/2 =-24.4 mV, z =4.2 e − . ( c ) Summary of the fraction of the peak current remaining after 10 ms for Nav1.4 and Nav1.4-WCW (mean±s.e.m.). *** t -Test, P <0.001. ( d ) Nav1.4-WCW whole-cell current responses to a steady-state inactivation protocol consisting of a 20 ms test pulse to −20 mV to assay the fraction of available (that is, non-slow inactivated) channels after a 1 s preconditioning pulse from −80 to 0 mV at room temperature (see inset). Holding potential was –120 mV and a 1 ms hyperpolarizing pulse to −140 mV preceded each test pulse. ( e ) The normalized peak current response during the test pulse is plotted against the voltage during the preconditioning pulse for five cells (open circles, mean±s.e.m., n =5) fit with a single Boltzmann plus an added constant (solid line; V 1/2 =-29.9 mV, z =4.9 e − , constant=0.27). The G–V relation for Nav1.4-WCW from b is shown inverted for comparison (dashed line). Full size image Nav1.4-WCW right-shifted the peak conductance–voltage (G–V) relation compared with Nav1.4 by 8 mV ( Fig. 1b ). Reversal potentials were not different (mean±s.e.m. ; Nav1.4: V rev =59.4±3.9 mV, n =5; Nav1.4-WCW: V rev =56.2±3.0 mV, n =8), suggesting that the relative permeabilities of Na + versus K + were unchanged. However, interpretation of the G–V is complicated by the fact that peak conductance for Nav1.4-WCW is a relatively steady-state measure, whereas the peak response for Nav1.4 is not at equilibrium. Although fast inactivation is largely abolished, slow inactivation remains intact in Nav1.4-WCW [28] . However, the onset of slow inactivation coincided almost exactly with the onset of channel activation during a 1 s preconditioning pulse ( Fig. 1d ). These data imply that Nav1.4-WCW channels do not inactivate at potentials too hyperpolarized to elicit channel activation, whereas wild-type sodium channels have been shown to fast inactivate from closed states before channel opening [30] . The coincidental removal of both fast inactivation following channel opening and inactivation from closed states suggests that the same fundamental mechanism may underlie these two processes. The above results are consistent with previous macroscopic observations for Nav1.4-WCW [28] , [29] . Subconductances in single Nav1.4 and Nav1.4-WCW channels Consistent with a lack of fast inactivation, single Nav1.4-WCW channels (nine patches) opened repeatedly throughout 200–400 ms depolarizing voltage steps from −60 to 0 mV ( Fig. 2a ). In contrast, single Nav1.4 channels (six patches) opened 1.5±0.2 times at all voltages tested before entering an absorbing closed state, which we attributed to inactivation. Currents obtained by averaging single channel records were reflective of macroscopic whole-cell current responses, suggesting that the observed single channel activity is representative of the channel’s behaviour ( Fig. 2b ). 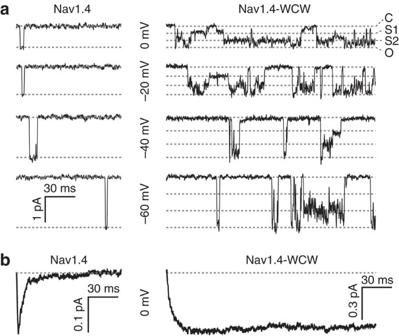Figure 2: Multiple conductance levels during gating of single Nav1.4-WCW channels. (a) Single channel records in response to 200 ms depolarizing pulses from −60 to 0 mV (−120 mV holding) for Nav1.4 (left, only first 100 ms shown) and Nav1.4-WCW (right) channels at 10 °C (filtered at 1 kHz for display). Dashed lines indicate observed conductance levels (C=closed, S1, S2, O; openings are downward). (b) Macroscopic responses obtained by averaging single channel records. Figure 2: Multiple conductance levels during gating of single Nav1.4-WCW channels. ( a ) Single channel records in response to 200 ms depolarizing pulses from −60 to 0 mV (−120 mV holding) for Nav1.4 (left, only first 100 ms shown) and Nav1.4-WCW (right) channels at 10 °C (filtered at 1 kHz for display). Dashed lines indicate observed conductance levels (C=closed, S1, S2, O; openings are downward). ( b ) Macroscopic responses obtained by averaging single channel records. Full size image Nav1.4-WCW single channel records exhibit multiple conductance levels, with subconductances at ~1/3 (S1) and 2/3 (S2) of the fully open (O) level ( Fig. 2a , Supplementary Fig. S2a ). On the basis of the frequent occurrence of events that within our resolution appear to transition directly between closed and fully open states (C↔O), or skip an intermediate level such as C↔S2 or O↔S1, and the similar conductance in O (17.5±1.4 pS) to that of Nav1.4 (17.1±1.4 pS), we conclude that these events represent subconductances in a single channel. The alternative, that the three conductance levels reflect coincidental opening of one to three low-conductance channels, would require a mechanism for cooperativity between channels to account for the frequent simultaneous opening and closing of two or three channels (within our resolution, channels appeared to open directly to the fully open state about 50% of the time at all voltages tested). Nav1.4 channels also exhibited a subconductance at ~1/2 of the main conductance level ( Supplementary Fig. S2a ). However, Nav1.4 subconductance events occurred infrequently, possibly because rapid inactivation limits the opportunity to visit a subconducting state, and thus precluded a more detailed kinetic analysis. To address the kinetics of individual conductance levels in Nav1.4-WCW, we idealized single channel records using the segmental k-means algorithm in the QuB software suite [31] allowing for two subconducting states ( Supplementary Fig. S2b ; see Methods). The presence of a single channel was determined by a lack of any visible stacked openings above the fully open level. Given their high probability of being open at −20 and 0 mV, this approach is a robust method for detecting patches containing single Nav1.4-WCW channels. The idealized conductance levels were representative of Gaussian fits to single channel amplitude distributions ( Fig. 3a ). Similar conductance levels were observed during deactivation of single Nav1.4-WCW channels ( Supplementary Fig. S3 ). Each conductance level displayed a linear current–voltage relation ( Fig. 3b ), with similar extrapolated reversal potentials ( Fig. 3c ). However, reversal potentials obtained by extrapolation of linear fits as shown in Fig. 3b are unlikely to detect <2-fold changes in Na + :K + permeability as observed for subconductances in Shaker potassium channels [32] . 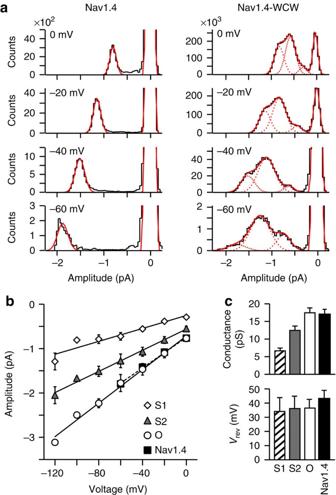Figure 3: Voltage dependence of individual conductance levels. (a) Single channel amplitude distributions for Nav1.4 (left) and Nav1.4-WCW (right). Histograms were obtained from all points in a single channel patch after discarding points adjacent to changes in amplitude in the idealized record to remove artifacts due to filtering. Red dashed lines are individual Gaussian fits to each conductance level, and the solid red line is their sum. (b) Current–voltage (I–V) relation for each conductance level (mean±s.e.m.) and its linear fit. The main conductance level for Nav1.4 (squares) nearly overlaps that of Nav1.4-WCW (circles). Data between −120 and −80 mV are from deactivation to the indicated potential (Supplementary Fig. S3). (c) Summary of the conductance (top) and reversal potential (Vrev, bottom) for each conductance level from linear fits to the I–V for individual patches. Conductances were (mean±s.e.m.), for Nav1.4-WCW: S1=6.8±0.9 pS, S2=12.5±1.3 pS, O=17.5±1.4 pS; and for Nav1.4: 17.1±1.4 pS. Extrapolated reversal potentials were (mean±s.e.m.), for Nav1.4-WCW: S1=34.2±9.9 mV, S2=36.3±8.9 mV, O=36.6±6.3 mV; and for Nav1.4: 43.4±5.8 mV. Figure 3: Voltage dependence of individual conductance levels. ( a ) Single channel amplitude distributions for Nav1.4 (left) and Nav1.4-WCW (right). Histograms were obtained from all points in a single channel patch after discarding points adjacent to changes in amplitude in the idealized record to remove artifacts due to filtering. Red dashed lines are individual Gaussian fits to each conductance level, and the solid red line is their sum. ( b ) Current–voltage (I–V) relation for each conductance level (mean±s.e.m.) and its linear fit. The main conductance level for Nav1.4 (squares) nearly overlaps that of Nav1.4-WCW (circles). Data between −120 and −80 mV are from deactivation to the indicated potential ( Supplementary Fig. S3 ). ( c ) Summary of the conductance (top) and reversal potential ( V rev , bottom) for each conductance level from linear fits to the I–V for individual patches. Conductances were (mean±s.e.m. ), for Nav1.4-WCW: S1=6.8±0.9 pS, S2=12.5±1.3 pS, O=17.5±1.4 pS; and for Nav1.4: 17.1±1.4 pS. Extrapolated reversal potentials were (mean±s.e.m. ), for Nav1.4-WCW: S1=34.2±9.9 mV, S2=36.3±8.9 mV, O=36.6±6.3 mV; and for Nav1.4: 43.4±5.8 mV. Full size image The S2 conductance often exhibited more noise than other levels, giving rise to the possibility that S2 may reflect the filtering of a rapid flicker from C↔O or S1↔O. To examine this possibility, we fit amplitude histograms from sojourns to S2 with beta distributions, which have been shown to describe amplitude histograms resulting from filtering of a flicker between two conductances [33] . However, it is difficult to conclusively determine whether this is the case as beta distribution and Gaussian fits were nearly indistinguishable ( Supplementary Fig. S4a ). If S2 does reflect a rapid flicker, then the estimated rate of flicker shows very little voltage dependence ( Supplementary Fig. S4b ). The WCW mutations do not disrupt channel activation The latency to first opening following depolarization onset was highly voltage-dependent for each individual conductance level, with more depolarized potentials eliciting channel opening faster on average ( Fig. 4a ). Although latencies to O and S2 were similar, on average the first event in S2 occurred slightly later than that in O. In contrast, latency to S1 was much longer than that for S2 or O. However, the voltage dependence of the weighted time constant from biexponential fits to the cumulative probability of having first opened was similar for each conductance level, suggesting that the set of closed states that is traversed in the activation pathway before reaching each conducting state have a similar voltage dependence ( Fig. 4c ). The probability of observing a null sweep (that is, no visible channel activity during the 200 ms pulse) was also voltage-dependent, decreasing from about 80% at −60 mV to 30% at 0 mV. 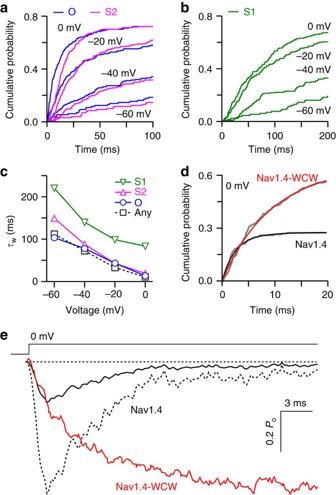Figure 4: Channel activation is not altered in Nav1.4-WCW. (a,b) Cumulative probability of first opening to each individual conductance level during activation from -60 to 0 mV (maximum probability increases with voltage). The reduction of the maximum from unity reflects the probability of observing a null sweep with no channel activity. Note expanded time scale inb. (c) Summary of the weighted time constants from biexponential fits to the cumulative probability of first opening for each individual conductance level and for opening to any level. (d) A comparison of the cumulative probability of first opening for Nav1.4 and Nav1.4-WCW during the first 20 ms of activation at 0 mV. Smooth lines are biexponential fits. (e) Comparison of the average single-channel response scaled to the observed peak open probability during activation at 0 mV for Nav1.4 (solid black) and Nav1.4-WCW (red). The response for Nav1.4 is also shown after normalizing to the peak response for Nav1.4-WCW (dotted black). Figure 4: Channel activation is not altered in Nav1.4-WCW. ( a , b ) Cumulative probability of first opening to each individual conductance level during activation from -60 to 0 mV (maximum probability increases with voltage). The reduction of the maximum from unity reflects the probability of observing a null sweep with no channel activity. Note expanded time scale in b . ( c ) Summary of the weighted time constants from biexponential fits to the cumulative probability of first opening for each individual conductance level and for opening to any level. ( d ) A comparison of the cumulative probability of first opening for Nav1.4 and Nav1.4-WCW during the first 20 ms of activation at 0 mV. Smooth lines are biexponential fits. ( e ) Comparison of the average single-channel response scaled to the observed peak open probability during activation at 0 mV for Nav1.4 (solid black) and Nav1.4-WCW (red). The response for Nav1.4 is also shown after normalizing to the peak response for Nav1.4-WCW (dotted black). Full size image During activation at 0 mV, the probability of having first opened increased with a similar time course for both Nav1.4 and Nav1.4-WCW up to the time of peak current in Nav1.4 ( Fig. 4d ). This suggests that the rate constants for activation are similar for Nav1.4 and Nav1.4-WCW. However, although Nav1.4 activation saturated within 10–20 ms at 0 mV, Nav1.4-WCW channels continued to open for the first time much later into the voltage step. For Nav1.4, these late openings are likely masked by inactivation from closed states before opening (that is, if the channel has not opened within ~20 ms of the depolarization, it is likely to already be inactivated). Thus, removing closed-state inactivation in Nav1.4-WCW ( Fig. 1d ) reveals a prolonged activation time course despite having little effect on the overall activation rate. Similar late channel activation was previously observed for other inactivation-deficient preparations including N1662A, another mutation that may reside within the inactivation gate [20] , and after treatment with NBA [25] . Scaling the average current responses for Nav1.4 and Nav1.4-WCW to their relative maximal open probabilities shows that their rising phases up to the time to peak for Nav1.4 are nearly indistinguishable ( Fig. 4e ). Peak open probabilities observed here are similar to previous reports of single Nav1.4 and inactivation-deficient sodium channel preparations [25] , [34] . These data show that the activation process in Nav1.4 can last much longer than the time to peak, where it is occluded by fast inactivation which can have a major role in shaping the rising phase of macroscopic currents [23] , [27] . As channels progress from closed to open to inactivated states, a right shift in the G-V with no change in the rate constants of activation suggests that Nav1.4-WCW speeds at least one backward rate along the deactivation pathway from open to closed states. This is consistent with the idea that deactivation involves pushing the inactivation particle out of its docking site, the energetic cost of which is absent for Nav1.4-WCW [35] . In other words, removal of energetic stabilization of the open state by binding of the inactivation particle may account for the rightward shift in the G–V curves. Consistent with this idea, the QQQ mutations right shift the G–V by 5 mV (ref. 8 ), and another mutation in the putative docking site for the inactivation particle, N1662A, also gives rise to late channel activation and right shifts the G–V by 10 mV (ref. 20 ). Dwell times in individual conductance levels Nav1.4-WCW dwell time distributions for each conductance level were fit with sums of exponentials by maximizing their log likelihood [36] ( Supplementary Fig. S5 , Supplementary Table S1 ). Closed times indicate the presence of at least three closed states, whereas dwells in O were well described by a single fully open state with similar open times to Nav1.4. Both subconductances were fit with a fast and slow component. However, the fast component was not well resolved, and is likely contaminated by filtering of brief events to other levels. Thus, we took the slow component as representative for dwells in S1 and S2, although this is an upper limit given any missed brief flickers. Bursting activity was defined as groups of openings separated by closures shorter than 5 ms. After first opening, most of the voltage dependence during Nav1.4-WCW channel activation could be attributed to the long closures between bursts which decreased in frequency and duration with increasing depolarization. Given the similar steep voltage dependence for the first latencies, it is possible that these long closures reflect a return to voltage-dependent closed states along the activation pathway. Dwell times in S1 were not very voltage-dependent, whereas openings to S2 and O increased in duration about two-fold from −60 to 0 mV. Thus, prolonged dwells in subconducting states contribute to an overall longer and voltage-dependent open time for Nav1.4-WCW compared with Nav1.4, which gives rise to periods of high open probability during bursting activity akin to observations in other inactivation-deficient preparations [25] , [34] , [37] , [38] . Kinetics of individual conductance levels The average probability in each conductance level ( P S1 , P S2 , P O ) was computed from the idealized records for every time point ( Fig. 5a ). P O increased rapidly early on during activation, whereas P S1 and P S2 increased more slowly. At 0 mV, P O exhibits a peak and subsequent slow decay. This slow decay could reflect either a small contamination in the observed activation process from slow inactivation, or a transition from O→S1/S2. In the latter case, we would predict that after opening, P O should decay with similar kinetics to a rise in P S1 or P S2 . To test this, we computed the conditional probability in each conductance level (CP S1 , CP S2 , CP O ) by averaging the probability at every time point after aligning each sweep to the time of first opening to any level ( Fig. 5b ). After first opening, CP O decays with a similar time course to a rise in CP S2 , suggesting that on average the pore first adopts a fully open conformation followed by a rearrangement associated with the S2 subconductance. In contrast, CP S1 does not show any obvious correlation with respect to the time of initial channel opening. Thus, S1 may represent an allosteric pore conformation off the main activation pathway. 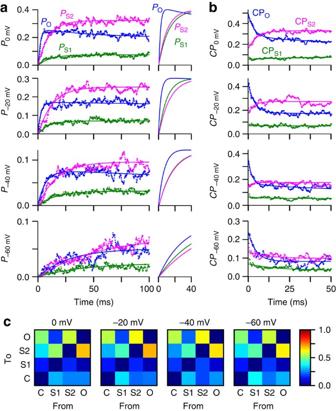Figure 5: Kinetics of individual conductance levels. (a) Average probability at every time point for each conducting state from idealized records (dots, only first 100 ms shown), and fits to the equation ΣiAi[1−exp(−t/τi)] (lines, seeSupplementary Table S2). The first 40 ms period is shown on the right after normalizing the fits to illustrate the relative kinetics of the initial rise in probability for each level. (b) Average conditional probability at every time point after aligning the idealized records so that the first event in each sweep occurs at time zero (dots), and fits to the equation ΣiAiexp(−t/τi)+ constant (lines, seeSupplementary Table S2). (c) The probability of transitioning between each conductance level during activation gating at each potential tested (0.5 ms resolution). Figure 5: Kinetics of individual conductance levels. ( a ) Average probability at every time point for each conducting state from idealized records (dots, only first 100 ms shown), and fits to the equation Σ i A i [1−exp(− t / τ i )] (lines, see Supplementary Table S2 ). The first 40 ms period is shown on the right after normalizing the fits to illustrate the relative kinetics of the initial rise in probability for each level. ( b ) Average conditional probability at every time point after aligning the idealized records so that the first event in each sweep occurs at time zero (dots), and fits to the equation Σ i A i exp(− t / τ i )+ constant (lines, see Supplementary Table S2 ). ( c ) The probability of transitioning between each conductance level during activation gating at each potential tested (0.5 ms resolution). Full size image Figure 5c shows the probability of an individual channel transitioning between conductance levels at 0.5 ms resolution. Approximately 50% of channel openings from the closed state occur directly to the fully open state, from which a channel will transition to the S2 subconductance about 70% of the time. Thus, the behaviour of single channels follows a preferential sequence of gating steps C→O→S2, consistent with the kinetics of the ensemble probability in each conductance level described above. Relationship between specific voltage sensors and the pore The kinetics of the probability in individual conductance levels from single molecules shows that the time course of the rise and subsequent decay (inactivation) in the open probability of Nav1.4 corresponds nearly exactly to the rate of entry into the O and S2 conductance levels in Nav1.4-WCW, respectively ( Fig. 6a ). However, unlike the inactivated state in Nav1.4, the S2 state is not absorbing, and therefore we do not observe a substantial decrease in P O with time (that is, channels reach an apparent equilibrium between O and S2). 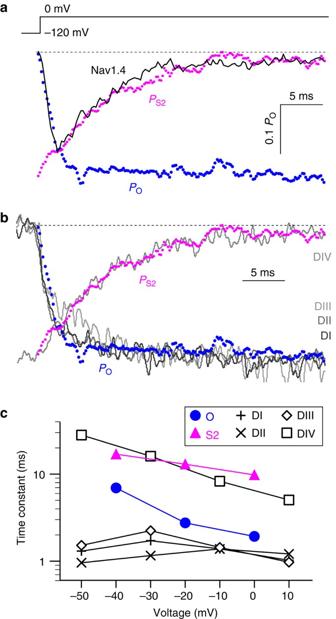Figure 6: Individual conductance levels are correlated with the movement of specific voltage-sensing domains. (a) Average single channel open probability for Nav1.4 during activation at 0 mV (black) overlaid with the probability for Nav1.4-WCW to be either fully open (PO, blue dots) or in a state associated with the S2 subconductance (PS2, magenta dots).PS2is shown inverted and scaled to illustrate its similar time course to that of Nav1.4 macroscopic inactivation. (b)POandPS2are shown as inaoverlaid with fluorescence signals from fluorophores attached to individual voltage sensors from domains I–IV in Nav1.4 (Supplementary Fig. S6). Because fluorescence signals were prohibitively difficult to reliably obtain below room temperature, these signals were uniformly scaled in time to account for the different temperatures at which the single channel (10 °C) and fluorescence (room temperature) were obtained (see methods). (c) Summary of the voltage dependence of the time constants for entry into the S2 and O conductance levels (seeFig. 5), and the fast time constant from exponential fits to the fluorescence responses from individual voltage-sensing domains (Supplementary Fig. S6), after scaling the fluorescence in time as described above. Figure 6: Individual conductance levels are correlated with the movement of specific voltage-sensing domains. ( a ) Average single channel open probability for Nav1.4 during activation at 0 mV (black) overlaid with the probability for Nav1.4-WCW to be either fully open ( P O , blue dots) or in a state associated with the S2 subconductance ( P S2 , magenta dots). P S2 is shown inverted and scaled to illustrate its similar time course to that of Nav1.4 macroscopic inactivation. ( b ) P O and P S2 are shown as in a overlaid with fluorescence signals from fluorophores attached to individual voltage sensors from domains I–IV in Nav1.4 ( Supplementary Fig. S6 ). Because fluorescence signals were prohibitively difficult to reliably obtain below room temperature, these signals were uniformly scaled in time to account for the different temperatures at which the single channel (10 °C) and fluorescence (room temperature) were obtained (see methods). ( c ) Summary of the voltage dependence of the time constants for entry into the S2 and O conductance levels (see Fig. 5 ), and the fast time constant from exponential fits to the fluorescence responses from individual voltage-sensing domains ( Supplementary Fig. S6 ), after scaling the fluorescence in time as described above. Full size image Given that the DIV voltage sensor has been implicated as having a unique role in inactivation [18] , we asked whether movement of specific voltage sensors could underlie distinct conductance levels. To test this, we measured fluorescence signals from fluorophores attached to individual voltage sensors in Nav1.4 during depolarizing steps ( Supplementary Fig. S6 ). Optical signals obtained at room temperature were uniformly scaled to account for the temperature difference between these and single channel measurements (see methods). Comparison of the kinetics of P O and P S2 with the relative time courses of fluorescent responses from individual voltage sensors shows that DI-III voltage sensors track entry into O, whereas the DIV voltage sensor tracks entry into S2 ( Fig. 6b ). This suggests that activation of voltage sensors in DI-III is correlated with formation of the fully open pore, whereas the S2 subconductance reflects a conformational state associated with inactivation and movement of the DIV voltage sensor. Subconductances represent distinct pore conformations Functionally, inactivation reflects entry into an absorbing closed state. Structurally, this is manifested as an occlusion of the pore upon binding of an intracellular hydrophobic motif [8] , [39] . This idea is supported by cysteine accessibility studies which show that cysteines introduced at sites such as F1579C become inaccessible during inactivation, but are orders of magnitude more accessible either before or upon removal of inactivation [40] . Given the correlation between the time course of S2 and Nav1.4 inactivation, we asked whether the subconductances observed here might simply reflect a weakly conducting form of inactivated state, where the inactivation motif still binds, but only partially occludes the pore. In this case, we predict that the partially bound inactivation motif should still pose a significant barrier to accessibility of larger reagents such as (2-(trimethylammonium)ethyl)methanethiosulfonate (MTSET) for sites normally hidden during inactivation. To test this, we examined the accessibility of an introduced pore cysteine (F1579C), which in a wild-type background shows no reactivity to internal MTSET while inactivated, but whose reactivity was shown to increase up to 50 M −1 s −1 upon impairing inactivation by changing the stimulus frequency and duration, or with a peptide toxin [40] . To avoid contamination from modification of L437C in WCW, we mutated position 437 to serine, hereafter referred to as WSW (L435W/L437S/A438W). Both Nav1.4-WSW and Nav1.4-WSW-F1579C severely disrupted fast inactivation similar to Nav1.4-WCW, suggesting that these mutations did not alter the overall behaviour of the WCW mutant ( Fig. 7a ). Exposure of Nav1.4-WSW-F1579C to 250 μM internal MTSET at 0 mV (see methods) conferred a gradual reduction in peak current amplitude with a second-order rate constant for modification of 5 360±180 M −1 s −1 , whereas no apparent modification of Nav1.4-WSW was observed ( Fig. 7b ). MTSET was unable to modify Nav1.4-WSW-F1579C at −120 mV, suggesting that this site is accessible in the open, but not closed state ( Fig. 7c ). 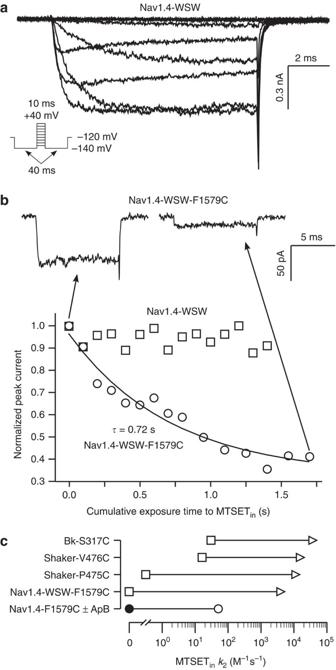Figure 7: The open pore of Nav1.4-WSW is fully accessible to internal MTSET. (a) Current responses to 10 ms voltage steps from −120 to 40 mV (20 mV steps) from a holding potential of −140 mV (see inset) from Nav1.4-WSW channels in inside–out patches excised from Xenopus oocytes. (b) The time course of the reduction in peak current for Nav1.4-WSW and Nav1.4-WSW-F1579C with respect to the cumulative exposure time to internal MTSET at 0 mV (see methods). Current responses for Nav1.4-WSW-F1579C before and after 1.7 s of exposure to internal MTSET at 0 mV are shown. (c) Second-order reaction rates of internal MTSET with Nav1.4-WSW-F1579C in the closed (square) and open (triangle) states. The reported change in closed to open state reaction rates for several residues in the pore of Shaker and BK potassium channels are shown for comparison41,42, as well as the reaction rate for Nav1.4-F1579C without (closed circle) and in the presence of the fast inactivation disrupting toxin Anthopleurin B (ApB) (open circle)40. Figure 7: The open pore of Nav1.4-WSW is fully accessible to internal MTSET. ( a ) Current responses to 10 ms voltage steps from −120 to 40 mV (20 mV steps) from a holding potential of −140 mV (see inset) from Nav1.4-WSW channels in inside–out patches excised from Xenopus oocytes. ( b ) The time course of the reduction in peak current for Nav1.4-WSW and Nav1.4-WSW-F1579C with respect to the cumulative exposure time to internal MTSET at 0 mV (see methods). Current responses for Nav1.4-WSW-F1579C before and after 1.7 s of exposure to internal MTSET at 0 mV are shown. ( c ) Second-order reaction rates of internal MTSET with Nav1.4-WSW-F1579C in the closed (square) and open (triangle) states. The reported change in closed to open state reaction rates for several residues in the pore of Shaker and BK potassium channels are shown for comparison [41] , [42] , as well as the reaction rate for Nav1.4-F1579C without (closed circle) and in the presence of the fast inactivation disrupting toxin Anthopleurin B (ApB) (open circle) [40] . Full size image The accessibility of F1579C in the Nav1.4-WSW non-fast inactivating background is comparable to the accessibility at homologous positions in Shaker and BK potassium channels in their fully open states [41] , [42] , and over two orders of magnitude faster than the accessibility of 1579C in a wild-type background even in the presence of Anthopleurin B toxin, which substantially impairs fast inactivation [40] ( Fig. 7c ). These data indicate that Nav1.4-WSW-F1579C is fully accessible to polar methanethiosulfonate compounds when the pore is open, consistent with the idea that the pore is not partially occluded by an inactivation motif, and that the subconductances observed here reflect distinct conformations of the open pore. Indeed, the subconductances may reflect pore conformations normally adopted during fast inactivation in wild-type channels. Despite the success in developing detailed quantitative models of potassium channel function in the absence of fast inactivation, studies of inactivation-deficient sodium channel preparations have yet to reveal a consistent picture of the activation process, in part due to a lack of robustly expressing inactivation-deficient mutants. Recently, Wang and coworkers [28] showed that Nav1.4-WCW eliminates macroscopic fast inactivation, while retaining similar conductance–voltage relationships to wild type. A similar Nav1.5 mutant retains the ability to bind an intracellular KIFMK peptide, indicating that these mutations prevent the native fast inactivation motif from accessing its docking site [43] . Removing inactivation by protein engineering overcomes the limitations of exogenous applications but, similar to any other mutation-based study, it must be established that the mutation does not have other effects on channel gating. As shown by Aldrich et al., [23] for sodium channels, macroscopic current recordings cannot accurately estimate activation kinetics because of our inability to scale the peak currents correctly. Peak current is determined by both activation and inactivation, which occur at overlapping voltages. A more stringent measure of activation kinetics is the latency for single channels to open for the first time in response to a stimulus [23] , which are almost identical for Nav1.4 and Nav1.4-WCW ( Fig. 4d ). Furthermore, single channel measurements provide ensemble kinetics that are correctly scaled to the peak open probability, which show that macroscopic current rise for Nav1.4 and Nav1.4-WCW virtually superimpose up to the time to peak in Nav1.4 ( Fig. 4e ). Taken together, these findings establish that the WCW mutant has a limited, if any, effect on the activation gating. Apart from a lack of fast inactivation, the other notable functional difference between Nav1.4 and Nav1.4-WCW is the frequent occurrence of subconductances. Disrupting inactivation in sodium or potassium channels often reveals subconductances [32] , [37] , [44] , [45] , [46] , [47] . Single channel studies show that subconductances are also present, albeit at a lower frequency, in wild-type sodium [37] , [45] , [48] , [49] and Shaker potassium channels [50] , as well as other voltage-gated ion channels such as BK channels [51] . We also observed infrequent subconductance events during Nav1.4 gating ( Supplementary Fig. S2 ). These observations suggest that subconductances are an intrinsic aspect of sodium channel gating typically occluded by fast inactivation. Consistent with this idea, multiple lines of evidence suggest that the major features of the native pore remain unchanged in Nav1.4-WCW. For example, the conductance of the fully open state in Nav1.4-WCW is identical to Nav1.4 with very similar open times, suggesting that the mutant pore adopts a conformation similar to that of wild type. This is also supported by accessibility measurements, which show that its open-state accessibility to MTSET is comparable to that of a fully open potassium channel ( Fig. 7c ). Also, Nav1.4-WCW binds local anaesthetics such as lidocaine with similar affinity to wild-type [29] . The subconductances reported here for Nav1.4-WCW are long-lived and preferentially visited following channel opening to the fully open level. The relative kinetics of the probability in O and S2 are correlated with activation of the DI-III and DIV voltage sensors, respectively, with S2 and DIV also being correlated with fast inactivation in Nav1.4 over a range of voltages where channels are beginning to activate ( Fig. 6 ). These data indicate a mechanism underpinning coupling between DIV movement and fast inactivation [11] , [15] , [18] , [19] , [20] , [21] , [22] . We propose that DIV voltage sensor activation promotes a rearrangement of the pore to a permissible conformation for rapid binding of the inactivation motif ( Fig. 8 ). This is in contrast to models where DIV movement either relieves a steric hindrance for binding of the inactivation motif without affecting the pore [52] or is directly involved in occluding the pore [1] . Our mechanism requires that channel gating involve a conducting conformation of the pore distinct from that of the fully open state, which directly precedes fast inactivation ( Fig. 8 ). We posit that in wild-type channels inactivation occurs rapidly from the S2 state, such that subconductances are rarely observed, but which are revealed upon destabilization of the inactivated state. In this model, the S2 conductance arises either from the S2 state itself, or from a rapid flicker between S2 and inactivated states. In either case, our data implies that the rate-limiting step to inactivation in wild-type channels is the formation of the S2 pore. 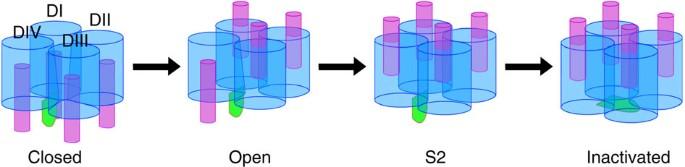Figure 8: Quasi-sequential activation model for sodium channel gating. A simple model depicting the preferential sequence of events during sodium channel activation. The closed to open transition represents all of the steps from resting to activated, and the S2 state represents a distinct conformation of the open pore, which precedes inactivation. In wild-type channels, inactivation occurs sufficiently rapidly from the S2 state so that it is rarely observed. For simplicity, the S1 subconductance is not included here, but this conductance may potentially be represented as a parallel set of states to indicate an independent allosteric conformation of the channel. In this model, inactivation from closed states proceeds via a transition from closed to S2. Figure 8: Quasi-sequential activation model for sodium channel gating. A simple model depicting the preferential sequence of events during sodium channel activation. The closed to open transition represents all of the steps from resting to activated, and the S2 state represents a distinct conformation of the open pore, which precedes inactivation. In wild-type channels, inactivation occurs sufficiently rapidly from the S2 state so that it is rarely observed. For simplicity, the S1 subconductance is not included here, but this conductance may potentially be represented as a parallel set of states to indicate an independent allosteric conformation of the channel. In this model, inactivation from closed states proceeds via a transition from closed to S2. Full size image The existence of a distinct preinactivated pore conformation can explain how both microscopic activation and inactivation rates are rapid while macroscopic current inactivation is slow, as the latter is limited primarily by the rate of entry into S2. Therefore, DIV mutations that disrupt the stability of the S2 state without affecting upstream activation or the inactivation motif can produce defects in inactivation gating [14] . The S2 state also offers a potential explanation for why some inactivation-impaired preparations reveal a prolonged activation time course [25] , [27] , whereas others seem not to [24] , [26] . For example, destabilizing the inactivated state will uncover the S2 conductance, thereby giving rise to a prolonged increase in channel open probability, whereas inhibiting entry into S2 will also effectively remove inactivation without exhibiting additional conductances or a prolonged activation time course. Thus, prior apparently conflicting results may reflect differential effects of various perturbations that either inhibit formation of the pore conformation preceding inactivation or binding of the inactivation particle itself. In addition, preferential binding of anaesthetics such as lidocaine to the S2 pore conformation may explain apparently conflicting observations regarding the affinity of these drugs for open versus inactivated states [29] , [53] . A second open state was previously reported for squid axon sodium channels at depolarized potentials where inactivation is incomplete [54] . In this study, the lifetime of the first opening in a burst was distinct from subsequent openings, suggesting that the pore underwent a conformational change after first opening, similar to our proposed sequence of events ( Fig. 8 ). The occurrence of a second open-pore conformation immediately preceding pore block has also been observed in BK channels during block by an accessory beta2 subunit [55] . However, the second open state in squid axon sodium channels or the symmetric BK channel has not been associated with movement of an individual voltage sensor. In Shaker potassium channels, brief intermediate subconductances have been associated with slightly asynchronous movement of highly coupled pore subunits [32] , [50] , whereas subconductances in a mutant drk1 potassium channel have been shown to directly reflect the number of activated subunits [56] , [57] , analogous to reports that subconductances reflect the number of ligand-bound subunits in glutamate receptors [58] . Thus, an intriguing possibility is that sodium channel opening initially involves only pore domains I-III, and that the S2 conductance reflects activation of the fourth pore domain. Alternatively, it is possible that activation of the DI-III voltage sensors results in the concerted opening of all four pore domains, and that slower activation of the DIV voltage sensor confers a separate change elsewhere in the permeation pathway. In either case, we show that, at a fundamental level, asynchronous activation in eukaryotic voltage-gated sodium channels is not just limited to the voltage sensors, but extends to the central pore domain. Specifically, activation of the DIV voltage sensor confers a second conducting pore conformation whose formation is the mechanism coupling DIV voltage sensor movement to fast inactivation. By rapidly occluding the second open-pore conformation, fast inactivation essentially converts an intrinsically two-step pore-opening process into one that behaves functionally as a single pore-opening transition. Constructs The inactivation-deficient rat skeletal muscle clone WCW was gifted by Dr Ging Kuo Wang and Dr Sho-Ya Wang. This triple mutant was recloned in the rat Nav1.4 background with multiple silent mutations to facilitate cloning as first described in Muroi and Chanda [59] , as well as an additional silent mutation at N434 to remove a Mfe I cut site introduced by the L453W mutation. The mutation C437S was introduced in the WCW background with the QUICKCHANGE mutagenesis kit (Stratagene, CA) to obtain the WSW construct, and subcloned into pBSTA for expression in Xenopus oocytes. Mutations were verified by sequencing the entire cloning cassette from enzyme cut sites Mfe I to BsiW I. Heterologous expression in HEK-293 cells and oocytes HEK-293 cells (ATCC) were cultured in a 37 °C, 5% CO 2 incubator using MEM supplemented with 10% fetal bovine serum, 100 U.I. ml −1 Penicillin, 100 μg ml −1 Streptomycin, 1 × sodium pyruvate and 1 × nonessential amino acids (Invitrogen). Cells were transfected with 1–2 μg rat Nav1.4 or rat Nav1.4-WCW cDNA in the pBudCE4.1 vector (gift from Dr David Wagner) using Lipofectamine LTX (Invitrogen). Recordings were made 24–72 h after transfection. Recordings were also made from a HEK-293 cell line stably expressing the rat Nav1.4-WCW construct [29] . The media for the stable line was supplemented with 200 μg ml −1 Geneticin (G418, Invitrogen) to maintain a selective pressure for cells expressing the mutant construct. No qualitative differences were observed in either macroscopic or single channel behaviour between channels expressed in the stable line and the transiently transfected mutant. For cysteine accessibility studies, the α-subunit (Nav1.4-WSW and Nav1.4-WSW-F1579C) and β1-subunit (HEK-293 cells contain endogenous β1A [60] ) cDNAs were transcribed using the mMessage mMachine Kit (Ambion Inc., Austin, TX), and their RNAs injected into defolliculated Xenopus oocytes in a ~1:1 molar ratio. Electrophysiology Single channel data were acquired from inside–out patches excised from HEK-293 cells using an Axon Digidata 1400 digitizer and Axon 200B amplifier (MDS Analytical Technologies) with AxoGraph software (AxoGraph Scientific, Sydney, AU). Recordings were sampled at 100–250 kHz and low-pass filtered at 10 kHz. The pipette/extracellular solution was (in mM): 140 NaCl, 0.5 CaCl 2 , 10 HEPES, pH 7.4, and the bath/intracellular solution was (in mM): 100 CsF, 30 KCl, 10 EGTA, 10 HEPES, pH 7.4. Quartz pipettes (Sutter QF-150-75) coated with Silguard (Dow Corning Corp., Midland, MI) and having a tip resistance of 10-15 MΩ were used for low noise recordings, and additionally a custom electromagnetic shield made from tin foil was placed around the recording chamber. The bath temperature was held at 10±1 °C with a low noise peltier-driven temperature-controlled chamber (QE-1HC, CL-100 and TCM-1, Warner Instruments, LLC, Hamden, CT). For whole cell recordings we used boroscilicate pipets (World Precision Instruments, Inc., Sarasota, FL) with a tip resistance of about 2 MΩ. Whole-cell series resistance compensation was usually 90%. Single channel analysis Single channel records were digitally filtered at f c =2 kHz and resampled at 5 kHz for analysis. The rise time of the filter T r was estimated as T r =0.3/ f c =150 μs, and the dead time T d was set to 2.5 sample points ( T d =500 μs) [36] . For Nav1.4-WCW channels, idealized records containing four conductance levels (closed, open and two subconductances) were generated using the segmental k-means algorithm in the QUB software suite [31] . For Nav1.4 channels, idealized records were obtained using segmental k-means with two conductance levels (closed, open), and similar results were obtained with a half amplitude threshold crossing. Because the fast component in some of the observed dwell time distributions for Nav1.4-WCW approached the limits in our ability to idealize an event, the reported apparent dwell times are likely contaminated by events reflecting the time spent not in a single state, but a set of states (for example, a conducting state and a brief unresolved closed state). However, the average time-dependent probability was insensitive to the omission of brief events, and thus is representative of the channel behaviour. We tested for artifacts in the voltage dependence of the dwell times at each conductance level due to the idealization by taking idealized records at −40 and −60 mV, where our signal to noise is greatest and rescaling them and adding noise to simulate the same records at −20 and 0 mV. At a filter cutoff of 2 kHz this method gave similar dwell time distributions at all signal to noise ratios reflecting our recorded data between −60 and 0 mV, whereas filtering at higher bandwidths such as 5 kHz resulted in erroneous voltage-dependent dwell times for the same record at different signal to noise levels. Thus, we restricted our analysis to data filtered at 2 kHz. Fluorescence Optical signals were recorded from a modified cut-open oocyte setup after labelling with 10 μM tetramethylrhodamine (Invitrogen) as described by Muroi and Chanda [59] . Cysteines were introduced in individual voltage sensors at the same sites used previously by Chanda and Bezanilla [18] . Fluorescence was recorded at room temperature, as fluorescent responses at colder temperatures were quenched and lacked sufficient signal to noise to extract reliable kinetics. One possibility for reduced signal to noise is that the solubility of oxygen, which is a potent quencher of fluorescence, increases at lower temperatures. To account for the temperature dependence of sodium channel kinetics [61] , fluorescence responses were uniformly scaled in time by a factor of 5 in order to compare them with the single channel kinetics observed at 10 °C. This scaling factor was based on the temperature dependence of ON gating currents in both skeletal ( Supplementary Fig. S7 ) and cardiac sodium channels [61] , as well as the known correlation between the activation of domains I-III and macroscopic current rise for Nav1.4 (ref. 18 ). Cysteine accessibility Accessibility to internally perfused MTSET was examined in inside–out patches from Xenopus oocytes 4–5 days post injection after mechanical removal of the viteline layer. The pipette/extracellular solution was (in mM): 115 NaCl, 5 KCl, 2 CaCl 2 , 10 HEPES, pH 7.2 and the bath/intracellular solution was (in mM): 100 K Aspartate, 20 NaCl, 2.5 MgCl 2 , 2 EGTA, 10 HEPES, pH 7.2. Fresh MTSET was dissolved in the bath solution and kept on ice before each experiment. Patches were directly perfused in bath solution without MTSET except when indicated, where the solution was rapidly exchanged using a solenoid computer controlled valve for one containing MTSET. Modification was assayed with a 10 ms test pulse to 0 mV from a holding potential of −120 mV to get the peak current response, followed by 2 s at −120 mV, 100 ms at 0 mV (or 2 s at −120 mV) in the presence of 250 μM internal MTSET to allow modification in the open (or closed) state, and another 10 s at −120 mV. This cycle was repeated as necessary to obtain the reaction rate from a single exponential fit to the time course of peak current versus cumulative MTSET exposure time. Dividing the reciprocal of the rate constant by the concentration of MTSET yielded the apparent second-order rate constant for modification. How to cite this article: Goldschen-Ohm, M.P. et al . Multiple pore conformations driven by asynchronous movements of voltage sensors in a eukaryotic sodium channel. Nat. Commun. 4:1350 doi: 10.1038/ncomms2356 (2013).